Neonatal testosterone suppresses a neuroendocrine pulse generator required for reproduction The pituitary gland releases hormones in a pulsatile fashion guaranteeing signalling efficiency. The determinants of pulsatility are poorly circumscribed. Here we show in magnocellular hypothalamo-neurohypophyseal oxytocin (OT) neurons that the bursting activity underlying the neurohormonal pulses necessary for parturition and the milk-ejection reflex is entirely driven by a female-specific central pattern generator (CPG). Surprisingly, this CPG is active in both male and female neonates, but is inactivated in males after the first week of life. CPG activity can be restored in males by orchidectomy or silenced in females by exogenous testosterone. This steroid effect is aromatase and caspase dependent, and is mediated via oestrogen receptor-α. This indicates the apoptosis of the CPG network during hypothalamic sexual differentiation, explaining why OT neurons do not burst in adult males. This supports the view that stereotypic neuroendocrine pulsatility is governed by CPGs, some of which are subjected to gender-specific perinatal programming. Pituitary hormones are released in the blood stream in pulses. This mechanism is essential to prevent both secretory machinery fatigue and target tissue desensitization. Although early evidence suggested that secretory pulses mirror the intermittent bursts of electrical activity exhibited by hypothalamic neuroendocrine cells [1] , [2] , the mechanisms that produce this pulsatility remain poorly understood, and several non-competing hypotheses are proposed. For example, the ultradian hourly rhythm in the activity of the hypothalamo–pituitary–adrenal axis may primarily reflect sub-hypothalamic endocrine feedforward–feedback mechanisms [3] . At variance, the pulsatility in the hypothalamo–pituitary–gonadal axis may in part involve the intrinsic oscillatory properties of the neuroendocrine gonadotropin-releasing hormone (GnRH)-producing cells [4] . In a different vein, the episodic pattern of release of the pituitary growth hormone may be caused by the alternate activity of the stimulatory and the inhibitory neuroendocrine cells secreting growth hormone-releasing hormone and somatostatin, respectively [5] , [6] . Underlying the notion of interacting hypothalamic neural networks driving pituitary activity is the concept of ‘neuroendocrine pulse generators’, or ‘visceromotor pattern generators’ as recently expanded by a proposal [7] regarding organizational principles of hypothalamic periventricular structures. However, electrophysiological evidence for non-circadian hypothalamic pacemakers remains scant [8] , [9] , despite early reports of oscillatory activity in cultured hypothalamic neurons [10] . Here we unveil such oscillatory activity by studying neuroendocrine magnocellular oxytocin (OT) neurons in rat anterior hypothalamic slices stabilized in an organotypic culture for several weeks. In these cultures, OT neurons display the typical coordinated electrical activity in bursts of action potentials (APs) [11] , [12] , [13] that in vivo provokes the intermittent secretion of neurohormonal pulses necessary for parturition and the milk-ejection reflex [14] . We have deciphered the origin of the bursting activity and questioned its link to the female-specific function of supraoptic OT neurons by evaluating how this activity conforms to mechanisms of sexual differentiation sculpting neural systems in the developing brain [15] . Our results suggest that this stereotypic pulsatility of OT neurons is entirely driven by a female-specific periventricular central pattern generator (CPG). A single CPG network specifically drives all the OT neurons We previously established that in organotypic cultures from postnatal day 5 (P5; birth=P1) females, all OT neurons burst concomitantly via a glutamatergic synaptic drive [11] , [12] , [13] . Here an AP-autocorrelation analysis applied to the raw recordings from OT neurons evidenced that these bursts were randomly superimposed on a background of rhythmic activity with a lower amplitude ( Fig. 1a–c,e ). The rhythmic discharge of OT neurons was not a result of intrinsic properties of these cells ( Fig. 1d,e ) and was coordinated among OT neurons that have no electrical or synaptic coupling ( Fig. 1f ; Supplementary Fig. 1 ). Taken with our previous demonstration [12] of spike-to-spike coincidence in the on-going activity in paired-recorded OT neurons, the present results clearly indicate that one single CPG network drives all the OT neurons simultaneously to ensure the physiological functions that perpetuate the species. The regularity of OT bursting was strongly modulated by GABAergic inputs and the sustained blockade of GABA A -receptors by bicuculline-induced robust oscillations made of bursts similar to those occurring spontaneously ( Fig. 1c,e,g ). This suggests that these neuromodulatory inputs are crucial for the adaptation of the neuroendocrine CPG network to incoming sensory (and hormonal) inputs, a feature shared by several motor CPGs [16] . In contrast, cognate magnocellular vasopressin (VP) neurons typically had an unsynchronized activity ( Supplementary Fig. 1b,c ) like in vivo [14] and their phasic activity depended on a glutamatergic [17] CPG that was essentially unresponsive to bicuculline ( Fig. 1h ). This suggests that in our cultures OT neurons are under the constant drive of a specific CPG network (OT–CPG). 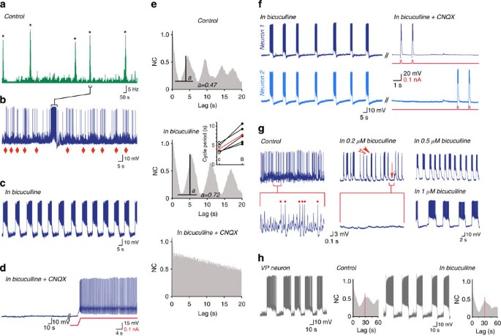Figure 1: Bursting activity in OT neurons is driven by a central pattern generator. (a) Rate metre of the activity of an OT neuron exhibiting spontaneous bursts (asterisks) in culture (P5 female). (b) Raw activity of the same OT neuron recorded in the current clamp mode; note the strong bursting (bracket) and the background rhythmic activity (red diamonds added manually). (c) This OT neuron exhibited large and regular membrane potential oscillations during bath application of the GABAA-receptor antagonist bicuculline. (d) Following an additional application of the AMPA-kainate glutamatergic-receptor antagonist CNQX to the bath, the OT neuron was silent, and no voltage-dependent bursting properties were observed during a depolarizing current injection. (e) Autocorrelograms corresponding to the raw recordings (b–d) demonstrating a rhythmic pattern under control conditions (top) and during bicuculline application (middle), and the absence of rhythmic firing pattern during bath-applied bicuculline and CNQX; the quality of the OT rhythm was higher in the presence of bicuculline compared with control conditions (a=0.72 and 0.47, respectively); the mean cycling period (inset, red) was significantly longer (cversusb,P=0.00137; Student’st-test) during bicuculline application compared with control conditions (n=5 cells each one from a different culture). (f) Paired recording of OT neurons synchronously oscillating under bicuculline (left), driven by glutamatergic CNQX-sensitive inputs and uncoupled (right, the injection of two brief transmembrane 0.05 nA per 100 ms positive currents into either cell did not affect the other). (g) Releasing the whole organotypic culture from GABAA-mediated inhibition by increasing concentrations of bicuculline progressively transforms OT neurons’ irregular spiking activity (top, red dots denote individual action potentials) into regular bursts (bottom right) similar to those occurring spontaneously; note progressively forming bursts (arrowheads) whereas inter-burst activity is dampening (arrow). (h) The typical oscillatory activity of VP neurons (left) was essentially unaffected during bath application of bicuculline (right) (a=31 and 37, respectively; cycling period: 28.1 s and 28.4 s, respectively), only the frequency of intra-burst action potentials has been shown to increase (15.01±4.1 versus 20.6±5.6 Hz, mean±s.e.m., in control versus bicuculline,P=0.003377, Student’st-test,n=5 each; see also ref.17). Figure 1: Bursting activity in OT neurons is driven by a central pattern generator. ( a ) Rate metre of the activity of an OT neuron exhibiting spontaneous bursts (asterisks) in culture (P5 female). ( b ) Raw activity of the same OT neuron recorded in the current clamp mode; note the strong bursting (bracket) and the background rhythmic activity (red diamonds added manually). ( c ) This OT neuron exhibited large and regular membrane potential oscillations during bath application of the GABA A -receptor antagonist bicuculline. ( d ) Following an additional application of the AMPA-kainate glutamatergic-receptor antagonist CNQX to the bath, the OT neuron was silent, and no voltage-dependent bursting properties were observed during a depolarizing current injection. ( e ) Autocorrelograms corresponding to the raw recordings ( b – d ) demonstrating a rhythmic pattern under control conditions (top) and during bicuculline application (middle), and the absence of rhythmic firing pattern during bath-applied bicuculline and CNQX; the quality of the OT rhythm was higher in the presence of bicuculline compared with control conditions ( a =0.72 and 0.47, respectively); the mean cycling period (inset, red) was significantly longer ( c versus b , P =0.00137; Student’s t -test) during bicuculline application compared with control conditions ( n =5 cells each one from a different culture). ( f ) Paired recording of OT neurons synchronously oscillating under bicuculline (left), driven by glutamatergic CNQX-sensitive inputs and uncoupled (right, the injection of two brief transmembrane 0.05 nA per 100 ms positive currents into either cell did not affect the other). ( g ) Releasing the whole organotypic culture from GABA A -mediated inhibition by increasing concentrations of bicuculline progressively transforms OT neurons’ irregular spiking activity (top, red dots denote individual action potentials) into regular bursts (bottom right) similar to those occurring spontaneously; note progressively forming bursts (arrowheads) whereas inter-burst activity is dampening (arrow). ( h ) The typical oscillatory activity of VP neurons (left) was essentially unaffected during bath application of bicuculline (right) ( a =31 and 37, respectively; cycling period: 28.1 s and 28.4 s, respectively), only the frequency of intra-burst action potentials has been shown to increase (15.01±4.1 versus 20.6±5.6 Hz, mean±s.e.m., in control versus bicuculline, P =0.003377, Student’s t -test, n =5 each; see also ref. 17 ). Full size image Age and sex hormone status condition CPG activity Sexual dimorphism in the ability of OT neurons to burst emerged with increasing age of the animals at tissue harvest. A majority (>90%) of cultures from both males and females at P5-harboured bursting OT neurons, and this number remained unchanged in females through P12 ( P >0.1, χ 2 -test, for P5 females ( n =42 cultures) versus P7 ( n =14), P9 ( n =45) and P12 females ( n =9)). However, a sharp decline was observed in males from P7 onwards (P7=36%, P9=8.8% and P12=6%) ( P <0.001, χ 2 -test, for P7 males ( n =25 cultures) versus P5 females ( n =42) and P5 males ( n =65), and for P7 males ( n =25) versus P9 ( n =57) and P12 males ( n =17); Fig. 2a,b ). These results suggest that circulating testicular testosterone (T) silenced an inherently female neural function before harvest. Accordingly, orchidectomy at P5 restored the bursting of OT neurons in cultures harvested at P9 (8.8% in intact versus 92.3% in castrated) ( P <0.001, χ 2 -test, intact males ( n =57 cultures) versus castrated males ( n =26)). In females, daily injections of T (0.5 mg per 50 μl sesame oil, subcutaneous) from P5–P7 suppressed this activity of the OT neurons in cultures harvested at P9 (85% in control versus 10.5% in treated) ( P <0.001, χ 2 -test, control females ( n =45 cultures) versus treated females ( n =19)) ( Fig. 2a,b ). Thus, this effect of testicular T displayed three characteristic features. First, the effect occurred at a specific postnatal age, P7. Second, the effect was irreversible and was observed despite an absence of the hormone during subsequent days in vivo and weeks in vitro . Third, the effect was independent of the genetic sex of the animals. This triad is typical of the ‘organizational effects’ of gonadal steroids in the sexual differentiation of the brain [15] . 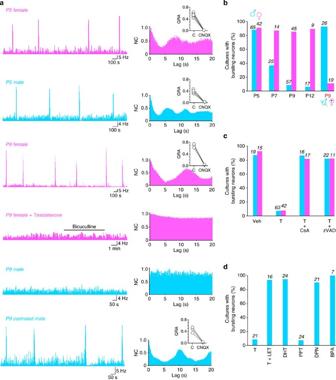Figure 2: Bursting activity is lost postnatally in males through pro-apoptotic sexual differentiation. (a) Left, Representative activity in OT neurons (as shown inFig. 1a, top) in cultures derived from age-matched (postnatal days 5 and 9), androgen-matched (normal P9 male and testosterone (T)-treated P9 female) and orchidectomized animals, showing how age and the androgen abolished both spontaneous bursting and bicuculline-induced oscillations (right, corresponding autocorrelograms; Quality of the Rhythmic Activity (QRA) plots show 3–5 individual cells each one from a different culture). (b) Effect of age, sex and T on the ability of OT neurons to burst (the number of cultures examined per group appears on top of bars); note the sharp decrease in males at P7 (P<0.001,χ2-test, for P7 males (n=25) versus P5 females (n=42) and versus P5 males (n=65), and for P7 males (n=25) versus P9 males (n=57) and versus P12 males (n=17)) and sex-reversal by orchidectomy and female androgenization (P<0.001,χ2-test, intact males (n=57) versus castrated males (n=26);P<0.001,χ2-test, control females (n=45) versus T-treated females (n=19)). All high-bursting groups (females and castrated males) were not statistically different (P>0.1,χ2-test), all low-bursting groups (P9 males, P12 males and T-treated females) were not statistically different (P>0.1,χ2-test). (c) Defeminization by T applied for the first 3 daysin vitroto tissues harvested from P5 animals was blocked by the apoptosis inhibitors cyclosporine A (CsA) and z-VAD-fmk to reach control vehicle (Veh) levels; note that there was no sex difference in response (males,P<0.001,χ2-test, for T alone (n=63) versus T+CsA (n=16) and versus T+zVAD (n=22); females,P<0.001,χ2-test, for T alone (n=42) versus T+CsA (n=17) and versus T+zVAD (n=11)). High-bursting groups (Veh, T+CsA and T+zVAD) were not statistically different (P>0.1,χ2-test). (d)In vitrodefeminization by T as incwas also blocked by aromatase inhibition with letrozole (LET) and was mimicked by the selective ERα agonist PPT; dihydrotestosterone (DHT), the selective ERβ agonist DPN and BPA had no effect (P<0.001,χ2-test, PPT (n=24) versus T+LET (n=16), versus DHT (n=24), versus DPN (n=21) and versus BPA (n=7)). High-bursting groups were not statistically different (P>0.1,χ2-test), low-bursting groups were not statistically different (P>0.1,χ2-test). Figure 2: Bursting activity is lost postnatally in males through pro-apoptotic sexual differentiation. ( a ) Left, Representative activity in OT neurons (as shown in Fig. 1a , top) in cultures derived from age-matched (postnatal days 5 and 9), androgen-matched (normal P9 male and testosterone (T)-treated P9 female) and orchidectomized animals, showing how age and the androgen abolished both spontaneous bursting and bicuculline-induced oscillations (right, corresponding autocorrelograms; Quality of the Rhythmic Activity (QRA) plots show 3–5 individual cells each one from a different culture). ( b ) Effect of age, sex and T on the ability of OT neurons to burst (the number of cultures examined per group appears on top of bars); note the sharp decrease in males at P7 ( P <0.001, χ 2 -test, for P7 males ( n =25) versus P5 females ( n =42) and versus P5 males ( n =65), and for P7 males ( n =25) versus P9 males ( n =57) and versus P12 males ( n =17)) and sex-reversal by orchidectomy and female androgenization ( P <0.001, χ 2 -test, intact males ( n =57) versus castrated males ( n =26); P <0.001, χ 2 -test, control females ( n =45) versus T-treated females ( n =19)). All high-bursting groups (females and castrated males) were not statistically different ( P >0.1, χ 2 -test), all low-bursting groups (P9 males, P12 males and T-treated females) were not statistically different ( P >0.1, χ 2 -test). ( c ) Defeminization by T applied for the first 3 days in vitro to tissues harvested from P5 animals was blocked by the apoptosis inhibitors cyclosporine A (CsA) and z-VAD-fmk to reach control vehicle (Veh) levels; note that there was no sex difference in response (males, P <0.001, χ 2 -test, for T alone ( n =63) versus T+CsA ( n =16) and versus T+zVAD ( n =22); females, P <0.001, χ 2 -test, for T alone ( n =42) versus T+CsA ( n =17) and versus T+zVAD ( n =11)). High-bursting groups (Veh, T+CsA and T+zVAD) were not statistically different ( P >0.1, χ 2 -test). ( d ) In vitro defeminization by T as in c was also blocked by aromatase inhibition with letrozole (LET) and was mimicked by the selective ERα agonist PPT; dihydrotestosterone (DHT), the selective ERβ agonist DPN and BPA had no effect ( P <0.001, χ 2 -test, PPT ( n =24) versus T+LET ( n =16), versus DHT ( n =24), versus DPN ( n =21) and versus BPA ( n =7)). High-bursting groups were not statistically different ( P >0.1, χ 2 -test), low-bursting groups were not statistically different ( P >0.1, χ 2 -test). Full size image Testosterone silences CPG activity at hypothalamic level To determine whether T acts locally in the hypothalamus, slices from P5 animals of both sexes were exposed to the hormone (10 −7 M) for the first 3 days of in vitro culture (3DIV), mimicking the in vivo treatment from P5 to P7. This exposure abolished the ability of OT neurons to burst in cultures from both male (89% in control versus 9% in treated) and female (93% in control versus 9.5% in treated) animals ( P <0.001, χ 2 -test, for control males ( n =19 cultures) versus T-treated males ( n =63) and for control females ( n =15) versus T-treated females ( n =42); Fig. 2c ), indicating a defeminization of the local networks. Apoptosis inhibitors block the action of testosterone Defeminization by T might involve neuronal apoptosis, which has been reported to occur in the anteroventral periventricular nucleus (AVPV). The AVPV projects to neuroendocrine GnRH neurons to control a female-specific function, ovulation, and contains more neurons in adult females than males due to the presence of pro-apoptotic neonatal T [18] . Two strategies that were shown [19] to block gonadal steroid-induced apoptosis in the AVPV in vitro were tested here. Hypothalamic slices from P5 animals were exposed for 3DIV to T together with either cyclosporine A (CsA), which blocks the formation of the permeability transition pore in mitochondria, or z-VAD-fmk, a pan-caspase inhibitor. After exposure, the OT neurons continued to burst in cultures from both male and female animals (T alone <9% versus T+blokers >82%) (cultures from males, P <0.001, χ 2 -test, for T alone ( n =63) versus T+CsA ( n =16) and versus T+zVAD ( n =22); cultures from females, P <0.001, χ 2 -test, for T alone ( n =42) versus T+CsA ( n =17) and versus T+zVAD ( n =11)) ( Fig. 2c ). This finding indicates a rescue of pivotal target neurons that are likely to be upstream of OT neurons, similar to the case in the AVPV–GnRH circuit. The immunohistological analysis of the supraoptic nuclei of gonadally intact neonates at P5–9 and P12 revealed no sex difference in OT neuron numbers and a minimal number of apoptotic-like cell nuclei identified by Hoechst labelling ( n =four rats per sex per age, P >0.05, two-way analysis of variance (ANOVA), no effect of age or sex). An extended group of P7 animals was examined to capture any transient events that likewise revealed no sex difference ( n =15 rats per sex, P >0.05, Student’s t -test; Fig. 3 ). This result is consistent with previous report of an absence of sex difference in cell numbers in the supraoptic nucleus in adult rats [20] . This is also consistent with the model of a secretomotor OT neuron driven by a sexually dimorphic CPG. 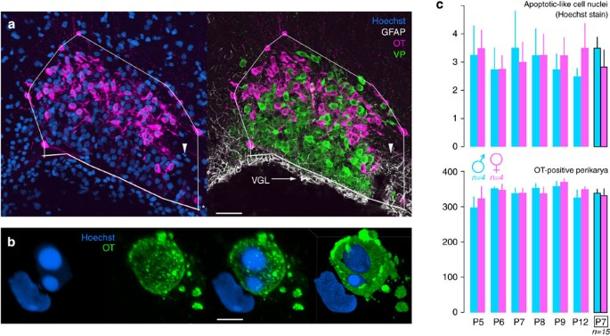Figure 3: Absence of significant cell death in the postnatal SONin vivo. (a) A quadruple-labelled section (as indicated) through the SON of a P5-male rat showing how the tissue was sampled for cell counts (arrowhead, typical apoptotic-like cell nucleus, as usually observed in peripheral SON). (b) 3D reconstruction of an apoptotic OT neuron from a different section demonstrating the efficiency of our procedures for detecting such rare events. (c) We observed no significant difference in numbers (mean±s.e.m.) of either Hoechst-stained fragmented cell nuclei (top) or OT-immunoreactive cell profiles (bottom) between the sexes; the numbers of animals are as shown; the groups of four were analysed by two-way ANOVA and the additional P7 groups of 15 were analysed by Student’st-test; top, no effect of age (P=0.979), no effect of sex (P=0.670), no age by sex interaction (P=0.966) and no sex difference were detected with the Student’st-test (P=0.716); bottom, no effect of age (P=0.517), no effect of sex (P=0.138), no age by sex interaction (P=0.855) and no sex difference were detected with Student’st-test (P=0.638). Out of the 26,616 OT-ir neurons counted, only 6 showed a fragmented nucleus (0.0002%). Micrographs shown are confocal stacks: (a)z=3.04 μm and scale bar, 100 μm, (b)z=7.33 μm and scale bar, 5 μm. VGL, ventral glial limitans; *, optic tract margin. Figure 3: Absence of significant cell death in the postnatal SON in vivo . ( a ) A quadruple-labelled section (as indicated) through the SON of a P5-male rat showing how the tissue was sampled for cell counts (arrowhead, typical apoptotic-like cell nucleus, as usually observed in peripheral SON). ( b ) 3D reconstruction of an apoptotic OT neuron from a different section demonstrating the efficiency of our procedures for detecting such rare events. ( c ) We observed no significant difference in numbers (mean±s.e.m.) of either Hoechst-stained fragmented cell nuclei (top) or OT-immunoreactive cell profiles (bottom) between the sexes; the numbers of animals are as shown; the groups of four were analysed by two-way ANOVA and the additional P7 groups of 15 were analysed by Student’s t -test; top, no effect of age ( P= 0.979), no effect of sex ( P= 0.670), no age by sex interaction ( P= 0.966) and no sex difference were detected with the Student’s t -test ( P= 0.716); bottom, no effect of age ( P= 0.517), no effect of sex ( P= 0.138), no age by sex interaction ( P= 0.855) and no sex difference were detected with Student’s t -test ( P= 0.638). Out of the 26,616 OT-ir neurons counted, only 6 showed a fragmented nucleus (0.0002%). Micrographs shown are confocal stacks: ( a ) z =3.04 μm and scale bar, 100 μm, ( b ) z =7.33 μm and scale bar, 5 μm. VGL, ventral glial limitans; *, optic tract margin. Full size image Testosterone acts via oestrogen receptor-α Localizing the targets of T requires a previous knowledge of the hormone’s active defeminizing form(s) and receptor(s), as multiple pathways may cooperate [21] . Therefore, hypothalamic slices from P5 males were exposed for 3DIV to T in combination with the aromatase inhibitor letrozole (LET), the non-aromatizable androgen receptor agonist dihydrotestosterone (DHT), the selective oestrogen receptor-α (ERα) agonist PPT (4,4′,4′′-(4-propyl-[1H]-pyrazol-1,3,5-triyl) trisphenol), the selective ERβ agonist DPN (2,3-bis(4-hydroxyphenyl)-propionitrile) or the endocrine disruptor bisphenol A (BPA), a weak ERα/β agonist (10 −7 M for all). LET blocked and PPT mimicked the action of T in a majority of cultures (PPT=8.3% versus all others >90.5%) indicating a single pathway through which intrahypothalamic aromatization of T into estradiol and ERα activation occurs ( P <0.001, χ 2 -test, PPT ( n =24 cultures) versus all others: T+LET ( n =16), DHT ( n =24), DPN ( n =21) and BPA ( n =7)) ( Fig. 2d ; Supplementary Fig. 2 ). This pattern is fully consistent with the broad ERα-dependent programme of apoptotic sexual differentiation of the rodent hypothalamus [21] whereby the freely circulating T in males, in contrast to the bound estradiol in females, is able to enter the brain for aromatization. Such a mechanism is also consistent with an action upstream of OT neurons that lack ERα [22] and aligns with our observation of an absence of sexual dimorphism in, and an effect of T on, the basic membrane properties and resting activity of OT neurons ( Fig. 4 ). 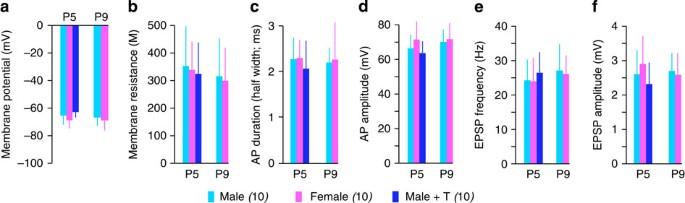Figure 4: Basic membrane properties and resting activity of cultured OT neurons are similar between sexes and across ages. There were no significant sex differences or changes after defeminization (P5 versus P9) or exposure to T of the slices harvested from P5 males (numbers are mean±s.e.m. ofn=10 cells per group, each cell from a different culture, the followingP-values refer to a comparison with P5 males by the non-parametric Kruskal–Wallis test). (a) Resting membrane potential: P5 male: −65.5±6 mV; P5 female: −68.8±5.6 mV (P=0.1220); P5 male+T: −63.7±3.7 mV (P=0.1570); P9 male: −66.8±6.1 mV (P=0.3269); P9 female: −68.9±7.1 (P=0.1457). (b) Membrane resistance: P5 male: 351.9±143.7 MΩ; P5 female: 338.9±103.0 MΩ (P=0.4106); P5 male+T: 322.8±114.27 MΩ (P=0.2952); P9 male: 315.3±138.5 MΩ (P=0.2896); P9 female: 299.5±120.0 MΩ (P=0.1886). (d) Action potential amplitude: P5 male: 66.3±8.0 mV; P5 female: 71.6±10.2 mV (P=0.1061); P5 male+T: 63.6±6.5 mV (P=0.1619); P9 male: 70.2±7.5 mV (P=0.1344); P9 female: 71.8±9 mV (P=0.0840). (c) Action potential duration (measured at half amplitude): P5 male: 2.25±0.47 ms; P5 female: 2.27±0.4 ms (P=0.4676); P5 male+T: 2.07±0.6 ms (P=0.2290); P9 male: 2.18±0.32 ms (P=0.3450); P9 female: 2.24±0.81 ms (P=0.4881). (e) EPSP frequency: P5 male: 24.1±6.15 Hz; P5 female: 23.9±6.7 Hz (P=0.1684); P5 male+T: 26.6±5.8 Hz (P=0.1983); P9 male: 27.4±7.7 Hz (P=0.1494); P9 female: 26.2±5.2 Hz (P=0.4135). (f) EPSP amplitude: P5 male: 2.6±0.7 mV; P5 female: 2.9±0.8 mV (P=0.1983); P5 male+T: 2.3±0.6 mV (P=0.1619); P9 male: 2.7±0.5 mV (P=0.1693); P9 female: 2.6±0.6 mV (P=0.4882). Figure 4: Basic membrane properties and resting activity of cultured OT neurons are similar between sexes and across ages. There were no significant sex differences or changes after defeminization (P5 versus P9) or exposure to T of the slices harvested from P5 males (numbers are mean±s.e.m. of n =10 cells per group, each cell from a different culture, the following P -values refer to a comparison with P5 males by the non-parametric Kruskal–Wallis test). ( a ) Resting membrane potential: P5 male: −65.5±6 mV; P5 female: −68.8±5.6 mV ( P =0.1220); P5 male+T: −63.7±3.7 mV ( P =0.1570); P9 male: −66.8±6.1 mV ( P =0.3269); P9 female: −68.9±7.1 ( P =0.1457). ( b ) Membrane resistance: P5 male: 351.9±143.7 MΩ; P5 female: 338.9±103.0 MΩ ( P =0.4106); P5 male+T: 322.8±114.27 MΩ ( P =0.2952); P9 male: 315.3±138.5 MΩ ( P =0.2896); P9 female: 299.5±120.0 MΩ ( P =0.1886). ( d ) Action potential amplitude: P5 male: 66.3±8.0 mV; P5 female: 71.6±10.2 mV ( P =0.1061); P5 male+T: 63.6±6.5 mV ( P =0.1619); P9 male: 70.2±7.5 mV ( P =0.1344); P9 female: 71.8±9 mV ( P =0.0840). ( c ) Action potential duration (measured at half amplitude): P5 male: 2.25±0.47 ms; P5 female: 2.27±0.4 ms ( P =0.4676); P5 male+T: 2.07±0.6 ms ( P =0.2290); P9 male: 2.18±0.32 ms ( P =0.3450); P9 female: 2.24±0.81 ms ( P =0.4881). ( e ) EPSP frequency: P5 male: 24.1±6.15 Hz; P5 female: 23.9±6.7 Hz ( P =0.1684); P5 male+T: 26.6±5.8 Hz ( P =0.1983); P9 male: 27.4±7.7 Hz ( P =0.1494); P9 female: 26.2±5.2 Hz ( P =0.4135). ( f ) EPSP amplitude: P5 male: 2.6±0.7 mV; P5 female: 2.9±0.8 mV ( P =0.1983); P5 male+T: 2.3±0.6 mV ( P =0.1619); P9 male: 2.7±0.5 mV ( P =0.1693); P9 female: 2.6±0.6 mV ( P =0.4882). Full size image The hypothalamic periventricular area and CPG activity The anatomical targets of T thus express both aromatase and ERα, which are two combined features of the neonatal periventricular area (PeV) [23] . In the neonatal PeV, ERα-positive cells are all neurons ( Figs 5a and 6a ); indeed, removing the PeV from hypothalamic slices harvested at P5, while without any effect on VP neurons, abolished the bursting activity of the OT neurons in the cultures of both sexes, that is, replicated the effect of T ( Fig. 5 ). Accordingly, histological analyses of the PeVs of gonadally intact male and female neonates at P5–9 and P12 revealed an on-going active apoptosis that slowed stepwise in both sexes with increasing age ( n =10 rats per sex per age; age groups P5, P6–7, P8–9 and P12 differed from one another, P <0.05, two-way ANOVA) ( Fig. 6b,c ). The incidence of cell death revealed by Hoechst staining of nuclear fragmentation showed no sex difference ( n =10 rats per sex per age, no effect of sex, P >0.05, two-way ANOVA; Fig. 6c ). In line with this, the segment of the PeV studied here has not appeared sexually dimorphic in adult rats [24] . The active cell death observed here may however affect in a commensurate manner, different networks in males and females, explaining the apparent sexual ‘neutrality’ of the PeV in adults. The incidence of cell death revealed by immunolabelling for an activated caspase 3 was comparatively much lesser ( Fig. 6c ). This suggests that caspase-dependent cell death is a minor component of the on-going morphogenesis, and/or that caspase activation is a short-lasting event, more difficult to observe than nuclear fragmentation [25] , [26] . Notwithstanding, this allowed to detect higher apoptotic rates in males, statistically significant at P5 but emerging as a trend at P7 ( n =10 rats per sex per age, effect of sex at P5 only, P <0.05, two-way ANOVA). Although this trend fits with the sex-reversal effect of the pan-caspase inhibitor z-VAD-fmk, and with the previous [27] demonstration by retrograde tracing in adult female rats of a direct projection from the PeV to the supraoptic nucleus, this also essentially suggests that the OT–CPG network is a dispersed neuronal sub-population in the heterogeneous PeV, likely resembling the dopaminergic A14 neuronal group ( Fig. 6a ). This A14 group appeared largely untouched by apoptotic processes ( Fig. 6c ), pleading for a selectivity of the on-going morphogenesis. Clearly however, the demonstration that a specific neuronal type of the PeV generates or contributes to the CPG activity recorded from the supraoptic OT neurons cannot be answered by the sole use of our present model. 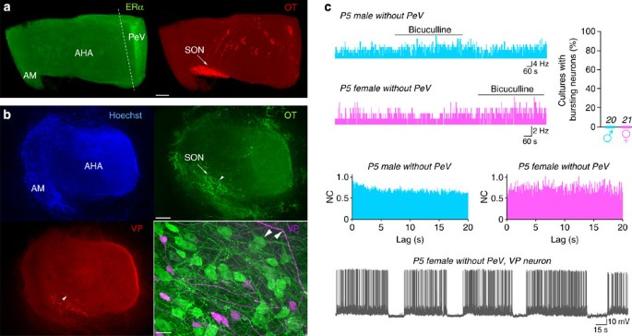Figure 5: The oestrogen-sensitive PeV is critical in burst generation. (a) A thick (350 μm) hypothalamic slice from a P5 male, representative of the tissue collected for organotypic culture, after paraformaldehyde fixation and immunolabelling for OT (red) and ERα (green); note the OT-rich SON (arrow) and the ERα-rich PeV, which was removed manually (dashed line) under binoculars before the culture. (b) PeV-excized organotypic culture, after 4 weeksin vitro, labelled for OT (green) and VP (red) and counterstained blue with Hoechst; note the anatomical preservation and healthy aspect of the neurons in the merged high magnification image (arrowheads point to the same elements). (c) In the PeV-excized cultures, spontaneous bursting activity and bicuculline-induced oscillations were never observed in OT neurons that had lost rhythmic drive, while the phasic activity in VP neurons was unaffected (compare withFigs 1and2). Scale bar, 200 μm ina, 500 μm and 50 μm (inset) inb. AHA, anterior hypothalamic area; AM, anterior amygdala. Figure 5: The oestrogen-sensitive PeV is critical in burst generation. ( a ) A thick (350 μm) hypothalamic slice from a P5 male, representative of the tissue collected for organotypic culture, after paraformaldehyde fixation and immunolabelling for OT (red) and ERα (green); note the OT-rich SON (arrow) and the ERα-rich PeV, which was removed manually (dashed line) under binoculars before the culture. ( b ) PeV-excized organotypic culture, after 4 weeks in vitro , labelled for OT (green) and VP (red) and counterstained blue with Hoechst; note the anatomical preservation and healthy aspect of the neurons in the merged high magnification image (arrowheads point to the same elements). ( c ) In the PeV-excized cultures, spontaneous bursting activity and bicuculline-induced oscillations were never observed in OT neurons that had lost rhythmic drive, while the phasic activity in VP neurons was unaffected (compare with Figs 1 and 2 ). Scale bar, 200 μm in a , 500 μm and 50 μm (inset) in b . AHA, anterior hypothalamic area; AM, anterior amygdala. 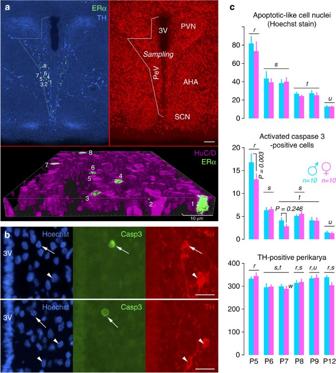Figure 6: Selective cell death in the postnatal PeVin vivo. (a) A triple-labelled section (as indicated) through the PeV of a P5-male rat shows the area sampled for cell counts based on the co-distribution of dopaminergic A14 group neurons (tyrosine hydroxylase (TH)-positive) with separate ERα-positive cells that are also positive for the neuronal marker HuC/D (as shown in the 3D reconstruction of a confocal stack through those cells, numbered 1–8). (b) Triple-labelled sections (as indicated) through the PeV of P5-male rats show (top) a TH-positive neuron with a fragmented nucleus and an activated Casp3-immunoreactivity, demonstrating the efficiency of our procedures in detecting such rare events, and (bottom) an unidentified Casp3-positive cell with a clearly fragmented nucleus (arrows and arrowheads point to the same apoptotic and healthy elements, respectively). (c) Selective cell death in the postnatal PeV; note the stepwise decline in numbers (mean±s.e.m.) of Hoechst-stained fragmented cell nuclei (top) and in the numbers of Casp3-positive cells (middle) but comparatively unchanged numbers of TH-positive dopaminergic A14 group neurons (bottom). No significant sex differences within age groups were observed, except at P5; at this age, the changes were detected through Casp3-labelling only. The numbers of animals are shown in italics (n=10 rats per sex per age). The analysis was performed by two-way ANOVA followed by the Student-Newman–Keulspost-hoctest with the significance level set atP<0.05; groups with different superscripts were significantly different. ANOVA results: top, no effect of sex (P=0.378), an effect of age (P<0.001) and no sex by age interaction (P=0.959); middle, no effect of sex (P=0.129), an effect of age (P<0.001) and no sex by age interaction (P=0.482); bottom, no effect of sex (P=0.567), effect of age (P=0.002) and no sex by age interaction (P=0.482). Out of 38,134 TH-ir neurons counted, only 7 displayed apoptotic-like features (0.0002%). Micrographs are video camera (a,c) or confocal (b,z=6.22 μm) images. AHA, anterior hypothalamic area; PeV, periventricular area; PVN, paraventricular nucleus; SCN, suprachiasmatic nucleus; 3V, third ventricle. scale bar, 100 μm inaand 20 μm inb. Full size image Figure 6: Selective cell death in the postnatal PeV in vivo . ( a ) A triple-labelled section (as indicated) through the PeV of a P5-male rat shows the area sampled for cell counts based on the co-distribution of dopaminergic A14 group neurons (tyrosine hydroxylase (TH)-positive) with separate ERα-positive cells that are also positive for the neuronal marker HuC/D (as shown in the 3D reconstruction of a confocal stack through those cells, numbered 1–8). ( b ) Triple-labelled sections (as indicated) through the PeV of P5-male rats show (top) a TH-positive neuron with a fragmented nucleus and an activated Casp3-immunoreactivity, demonstrating the efficiency of our procedures in detecting such rare events, and (bottom) an unidentified Casp3-positive cell with a clearly fragmented nucleus (arrows and arrowheads point to the same apoptotic and healthy elements, respectively). ( c ) Selective cell death in the postnatal PeV; note the stepwise decline in numbers (mean±s.e.m.) of Hoechst-stained fragmented cell nuclei (top) and in the numbers of Casp3-positive cells (middle) but comparatively unchanged numbers of TH-positive dopaminergic A14 group neurons (bottom). No significant sex differences within age groups were observed, except at P5; at this age, the changes were detected through Casp3-labelling only. The numbers of animals are shown in italics ( n =10 rats per sex per age). The analysis was performed by two-way ANOVA followed by the Student-Newman–Keuls post-hoc test with the significance level set at P <0.05; groups with different superscripts were significantly different. ANOVA results: top, no effect of sex ( P=0.378 ), an effect of age ( P<0.001 ) and no sex by age interaction ( P=0.959 ); middle, no effect of sex ( P=0.129 ), an effect of age ( P<0.001 ) and no sex by age interaction ( P=0.482 ); bottom, no effect of sex ( P=0.567 ), effect of age ( P=0.002 ) and no sex by age interaction ( P=0.482 ). Out of 38,134 TH-ir neurons counted, only 7 displayed apoptotic-like features (0.0002%). Micrographs are video camera ( a , c ) or confocal ( b , z =6.22 μm) images. AHA, anterior hypothalamic area; PeV, periventricular area; PVN, paraventricular nucleus; SCN, suprachiasmatic nucleus; 3V, third ventricle. scale bar, 100 μm in a and 20 μm in b . Full size image Our data show that CPG networks drive the sustained electrical activity displayed by neuroendocrine magnocellular hypothalamo-neurohypophyseal cells in vitro . This sustained activity, either in bursts of APs for OT neurons or phasic for VP neurons, is known in vivo to specifically allow the release of boluses of neurohormone into the blood stream [14] . The electrical activities of OT and VP neurons are quite similar in organotypic cultures and in vivo [17] , [28] , and the ability of OT neurons to burst in vitro fully recapitulates the known programme of sexual differentiation of the hypothalamus [15] . Thus, we likely provide here evidence for the existence of two separate neuroendocrine pattern (or pulse) generators [7] . It is thought that CPGs are building blocks of the central nervous system, not restricted to motor circuits, and can have a variety of architectures [16] . Clearly here, the CPGs driving OT and VP neurons in vitro differ in many aspects; in their anatomical location, that is, the PeV versus the wide surroundings of the SON [14] , respectively; in their rhythm; in their regulation by afferent inputs; last, in their developmental fate. It is therefore difficult to predict how the presently unveiled mechanisms apply to the other, parvicellular, neuroendocrine systems and their individual-specific ultradian rhythms. Another limitation is the paucity of available information concerning the in vivo activity of identified parvicellular neurons [29] and how this activity changes along with the occurrence of a secretory pulse of anterior pituitary hormones. Our results concerning the OT–CPG apparatus suggest that T eliminates a functional network during brain sexual differentiation. This is an unusual process, as evidence suggests that neurons typically die before establishing connections [15] , [18] , [19] , [30] . This finding raises the question of why the OT–CPG is spontaneously active in neonates. This may be because the OT neurons are actively contributing to neuroprotection around the time of birth [31] , [32] , [33] before switching to their sex-specific adult functions. In males, this switch requires shedding a neural apparatus that is inappropriate to the masculine brain-wiring programme, explaining why OT neurons have never been observed to burst in adult males. In females, that same autonomously active apparatus may later serve an additional purpose, for example, a neuroendocrine trophic function on reproductive target tissues [34] , [35] , before being silenced until the first parturition. This silencing, which currently receives no explanation, is also a feature of the developing gonadotropic axis [36] , [37] , the other component of the typically phasic reproductive function in the female sex. Presumably, this silencing may coincide with the reception of all of the developing afferents [38] that will integrate hormonal and sensory stimuli [39] to initiate appropriate activity to meet the specific physiological needs of labour and suckling. The present data do not allow conclusions about the architecture of the OT–CPG network. One unsolved mystery regarding the neuroendocrine control of the milk-ejection reflex is the coordination of the bursts in the entire population of OT neurons in both hemispheres during a secretory pulse [14] . In line with anatomical considerations [7] , our results suggest that there is one periventricular OT–CPG on each side of the brain, and that these CPGs are exquisitely sensitive to activity patterning by afferent inputs, a starting point for further in vivo investigations [39] . The defeminization of the OT–CPG is reminiscent of the similar developmental fate of the AVPV [40] , another hypothalamic periventricular ‘mullerian’ structure that is thought to entrain collective neurosecretory behaviour to trigger ovulation [18] . Our study thus expands on this by linking the morphogenetic action of a steroid hormone to the loss of the functionally defined output of a generator-effector system and thereby demonstrates how a neuroendocrine cell population acquires its specialized pulsatile capability from specifically organized afferent networks. Animals and surgical procedures Timed-pregnant, 10- to 12-week-old female Wistar rats (C.E.R.J., Le Genest Saint Isle, France) were received at G16 and were housed in our animal facility (lights on from 07:30–19:30 h). Dams were inspected three times daily, and litters from acknowledged parturitions were used. The day of birth was designated postnatal day 1 (P1), and litters were adjusted to ten pups on P2. Unless specified, all pups were intact subjects of the identified gonadal sex. Bilateral orchidectomies were performed under cryoanaesthesia on P5 through a small ventral midline incision that was subsequently sealed with liquid bandage (Laboratoires Urgo, France), and newborns were allowed to recover under heat. The sham animals were anaesthetized/incized/sealed only. T treatment of female newborns was a single subcutaneous injection given at 11:00–12:00 on P5, P6 and P7 at a dose (0.5 mg T propionate per 50 μl sesame oil, Sigma nos. T1875 and S3547) known to fully masculinize the hypothalamus [41] . The controls received oil only. All efforts were made to reduce the number of animals used and any distress caused by the procedures in accordance with the European Communities Council Directive of September 22, 2010 (2010/63/UE) and complying with the guidelines of INSERM and the local ethical comity of Bordeaux. Organotypic slice cultures Cultures from animals on P5, P7, P9 and P12 were investigated; the cultures from animals aged >P15 did not stabilize satisfactorily. These ages were chosen to clearly separate the developmental stages of sexual differentiation known to occur during critical periods with often-abrupt limits [42] . Cultures were prepared using the roller tube method [43] . Pups were anaesthetized with 5% isoflurane and decapitated. The brains were removed, blocked to the ventral hypothalamus/amygdala and coronally sectioned at 350 μm with a McIlwain tissue slicer. Two adjacent brain slices containing the supraoptic nucleus (SON) were selected within the anterior hypothalamus (posterior to the foramen of Monroe and anterior to the arcuate nucleus) and immersed in a Petri dish containing Gey’s solution (Eurobio no. CS1GEY0001, Courtaboeuf, France). The amygdalar region was removed lateral to the SON, and the slices were cut in halves along the third ventricle (see Fig. 5a ). Each half was placed on individual glass coverslips coated with heparinized chicken plasma (Cocalico no. 30-030-5L, Reamstown, PA, USA). Thrombin (Merck no. 112374) was added to coagulate the plasma and to allow the slice to adhere to the coverslip. The coverslip was inserted into a plastic flat-bottomed tube (Nunc no. 055054, Roskilde, Denmark) containing 750 μl of a medium consisting of 50% Eagle’s basal medium (Gibco no. 21540026, Fisher Bioblock, Illkirsh, France), 25% heat-inactivated horse serum (Gibco no. 26050088, Fisher Bioblock) and 25% Hanks balanced salt solution (HBSS; Gibco no. 24020091, Fisher Bioblock) enriched with glucose (7.5 mg ml −1 ) and 2 mM L-glutamine (Sigma no. G7513), pH 7.4 (290–295 mOsm). No antibiotics were used. The tubes were tightly capped, given a code number in our blinding strategy, inserted into a roller drum at 37 °C and rotated at ~15 turns h −1 . The medium was replaced twice per week. The cultures were allowed to flatten and stabilize for 4–10 weeks before electrophysiological recording became possible, at which time the anatomical organization was still discernible (see Fig. 5b and previous discussions of histofunctional issues [44] ). Drugs and hormones were applied in the culture medium in 1 μl of vehicle to achieve a final concentration of 0.1 μM. In experiments to block the action of T, the slice was first pre-incubated with the blocking agent (z-VAD-fmk, CsA or LET) alone for 2 h; then T propionate was added for 3 days, after which normal medium was used. This length of treatment over 3 days corresponds to the delay in the first changes in electrical activity observed in males from P5–P7. Control cultures received the vehicle only. The following hormones and drugs were all applied at 10 −7 M for the first 3 days in vitro : bisphenol A (>99% pure, Sigma), CsA (>98.5% pure, Sigma), DHT (5α-androstan-17β-ol-3-one, >97% pure, Sigma), DPN (Tocris Bioscience), LET (>98% pure, Sigma), PPT (Tocris Bioscience), T propionate (Sigma) and z-VAD-fmk (Caspase inhibitor I, Calbiochem). Electrophysiological recordings A culture was transferred from the incubator to a temperature-controlled chamber (34±0.2 °C) fixed to the stage of an inverted microscope (Diaphot, Nikon). SON magnocellular neurons were identified on the basis of their large size and their grouping away from a palisade of ependymocytes with beating cilia. The microelectrode was directed towards the cell to be recorded using oleic micromanipulators (Narishige). For recording, the culture was perifused (0.7 ml min −1 ) with Yamamoto's solution (in mM): NaCl (125), KCl (3), MgSO 4 (1), KH 2 PO 4 (1.25), NaHCO 3 (5), CaCl 2 (2), glucose (5) and HEPES (10); pH 7.25; 293–295 mOsm. Intracellular microelectrodes were pulled from borosilicate glass capillaries (OD: 1 mm, ID: 0.5 mm; Howard Happaratus) with a Flaming/Brown P87 puller (Sutter Instruments) and filled with 1 M potassium acetate containing 1% biocytin (Sigma). Electrode resistance varied from 150–250 MOhms. The intracellular potentials of the neurons were recorded through a single microelectrode using an Axoclamp-2A (Axon Instrument), which also permitted the injection of transmembrane currents (current clamp recording). Analyses of electrical activity Electrical signals were visualized on a digital oscilloscope (Tektronix TDS 2012B; Beaverton, OR, USA), recorded directly on a recorder (Gould thermal array recorder TA 11; Gould, Glen Burnie, MD, USA) and stored on a hard disk using pClamp 9 software (Axon Instruments) and a Digidata 1300 interface (Molecular Devices, Union City, CA, USA). The stored electrical activity was replayed, and sequential frequency histograms were calculated over 1-s integration periods and plotted versus time using an appropriate programme in pClamp 9. The data obtained from event analyses were compared statistically using the paired Student’s t -test (significance set at P <0.05). Because in an organotypic culture all OT neurons burst concomitantly [12] , a routine was used to discriminate neuronal activities in vitro . Thus, 1–4 subsequent neurons per culture were routinely recorded before ascribing a ‘bursting’ or a ‘non-bursting’ status to the OT neuronal population per culture. The results are expressed as numbers of bursting versus non-bursting cultures in each experimental group. Neurons displaying a membrane potential lower than −45 mV and an AP amplitude lower than 40 mV were discarded. Neurons that did not display spontaneous bursting activity after 15–20 min of recording were subjected to three phenotyping challenges. Either exogenous OT or bicuculline was applied to trigger bursts or oscillatory activity, respectively; if these approaches were inefficient, a hyperosmotic test (+25 mOsm) was administered to reveal phasic activity typical of vasopressinergic neurons [17] . On rare occasions these tests were negative, and triple-labelling immunocytochemistry was performed to reveal biocytin, OT and VP. Furthermore, an autocorrelation analysis (see Supplementary Fig. 3 ) was used to evaluate the periodicity as well as the regularity in neuronal activity [45] . Episodes of OT and VP neuron activity of 3–5 min in duration were analysed using custom scripts run within Spike2 software for Windows (CED, UK). Autocorrelograms were constructed from the spike trains of OT/VP cells converted to event times by setting a voltage threshold at half amplitude of APs. For each event, the numbers of events occurring in consecutive 0.1-s bins were counted over a 20-s time period for OT cells and 60-s time period for VP cells. This counting procedure was repeated for all events in the episodes of recorded activity, and the resulting counts were summed for each bin. The counts were normalized to the maximum bin count (that is, the first bin). This procedure produced a periodic function with decaying oscillations. The periodicity of the rhythmic activity was obtained by measuring the lags from time 0 to the second peak on autocorrelograms. Measuring the peak–to–trough amplitude of the second peak on autocorrelograms assessed the Quality of the Rhythmic Activity (QRA) of OT/VP cells. Its value (denoted a ) could potentially range from 0 to 1. A perfectly stable rhythm would have a QRA value of 1. Antibodies The primary antisera used were as follows: active (cleaved) caspase 3 (Casp3) (rabbit polyclonal, diluted 1:1,000; Millipore no. AB3623), ERα (rabbit polyclonal, 1:20,000; Millipore no. 06-935; Temecula, CA, USA), glial fibrillary acidic protein (chicken polyclonal, 1:1,000; US Biological no. G2032-25F; Swampscott, MA, USA), human neuronal protein HuC-HuD (HuC/D) (mouse monoclonal, clone 16A11, 1:750; Life Technologies no. A21272; Saint Aubin, France), OT [46] (mouse monoclonal to OT-associated neurophysin (OT–Np), clone PS38, 1:500; ATTC no. ATCCRL1950, Rockville, MD, USA; kind gift of Dr Harold Gainer, NIH, Bethesda, MD, USA), tyrosine hydroxylase (TH) (rabbit polyclonal, 1:3,000; Institut de Biotechnologies Jacques Boy No. 208020234; Reims, France) (mouse monoclonal, clone LNC1, 1:1,000; Millipore No. MAB318) (sheep polyclonal, 1:500, Pel-Freeze Biologicals No. P60101-0; Rogers, AR, USA) and VP (guinea-pig polyclonal, 1:800; Bachem No. T-5048; Bubendorf, Switzerland). When applied in cocktails, the anti-OT–Np and the anti-VP label essentially separated the neuronal populations ( Figs 3a and 5b ). Donkey IgGs conjugated to AMCA, DyLight 488, TRITC or DyLight 649 were used as secondary antisera (1:400; Jackson Immunoresearch Europe, Newmarket, Suffolk, UK). Immunocytochemical procedures Following our standard procedures [47] , the animals were overdosed with 20% chloral hydrate and perfused transaortically with 1–2 ml saline followed by 10–25 ml of a mixture of 4% paraformaldehyde and 0.2% picric acid in a 0.1 M phosphate buffer (pH 7.4). The brains were post-fixed in the same mixture for 24 h at 4 °C, cryoprotected overnight at 4 °C in a 0.1 M veronal buffer (VB; pH 7.4) containing 20% sucrose, embedded in Tissue-Tek (Sakura Finetek, Europe B.V., The Netherlands), frozen in liquid nitrogen and stored at −80 °C until use. The full rostrocaudal extent of the hypothalamus was cut into ten series of adjacent 12-μm-thick frontal cryostat sections collected on gelatinized slides (given a code number in our blinding strategy) and stored at −80 °C until use. Primary and secondary antisera were diluted in VB containing 0.25% Triton X-100 (Sigma) and applied at room temperature overnight and for 2 h, respectively. Streptavidin-Texas Red (1:200, Vector Labs. No. SA-5006; Eurobio/Abcys, Nanterre, France) was applied with the secondary antibodies. Organotypic cultures were fixed for 24 h as described above, rinsed in VB and processed in the same manner used for cryostat sections. The 350-μm-thick slices of the hypothalamus from the fresh tissue sectioner were fixed as described above and incubated at 4 °C for 5 days in primary antibodies (clone PS38, 1:2,000; rabbit anti-ERα 1:100,000) and for 24 h in secondary antibodies (1:1,000). Observation and acquisition were performed with epifluorescent (Zeiss Axiophot 1 equipped with a Leica DFC300X video camera; Carl Zeiss S.A.S., Le Pecq, France;) and confocal (Leica DMR TCS SP2 AOBS; Leica Microsystems France, Rueil-Malmaison, France) microscopes. Images were processed in Adobe Photoshop (Adobe Systems; San Jose, CA, USA) to permit correction for colour balance, brightness and contrast. Cell counts Cell death in the SON was examined at P5, P7, P9 and P12 (in one series of 9–10 sections per animal, four animals per sex). No sex difference was found, especially at P7, when the activity of the OT neurons changed in cultures of tissues from males. Because it is unclear how rapidly cell death may occur in vivo [26] , cell counts were extended to a larger group of P7 animals (for a total n =15 per sex) to ensure that no transient event had been overlooked. For both counting sessions, sections were double-labelled with anti-OT–Np revealed by DyLight 488-linked Donkey anti-mouse IgGs and the nuclear stain bisbenzimide (Hoechst. No. 33258, Cat. No. 14530, Fluka Chemie A.G., Ulm, Germany). Two parameters were chosen as indices of cell death. First, the number of OT–Np-immunoreactive (ir) cell bodies was evaluated. These cells were counted in the right hemisphere throughout the SON in confocal stacks of seven optical planes within the central 0.98 μm of the tissue sections. The optical planes had been separately acquired with a × 40 objective through the blue and green channels. Using ImageJ ( http://rsb.info.nih.gov/ij/ ), blue and green stacks were merged, and OT–Np-ir perikaryal profiles were manually selected on the basis of the presence of at least a rim of green cytoplasm around a section of blue nucleus ( Fig. 3a ). Exceptional instances of OT–Np-ir cell bodies with apoptotic-like nuclei were fully scanned using optimized Shannon–Nyquist sampling at × 63 and reconstructed in three dimensional (3D) with Imaris (Bitplane, St Paul, MN, USA) to ascertain their status ( Fig. 3b ). The second parameter estimated was the number of Hoechst-stained cell nuclei undergoing fragmentation/condensation [25] . These nuclei were counted bilaterally by direct inspection under an epifluorescence microscope at 40X and selected if located within the limits of the SON, as defined by the distribution of OT–Np-ir perikarya ( Fig. 3a ). The triggering of apoptosis ultimately results in the activation (cleavage) of caspases, including Casp3, the product of which can be detected by immunocytochemistry. This staining was performed here but not quantified by cell counts in the SON because of the very low occurrence of Casp3-ir cells in the SON. This finding is consistent with the very low number of apoptotic cell nuclei observed after Hoechst labelling. To quantify cell death in the PeV, series of sections (10–12 per animal) from the animals described above and from additional animals at P5, P6, P7, P8, P9 and P12 were used (in total, n =10 per sex per age). Sections were double-labelled for TH and Casp3 and counterstained with Hoechst ( Fig. 6b ). Counts were performed bilaterally by direct inspection under an epifluorescence microscope at × 40. Three indices of cell death were considered: first the number of apoptotic-like cell nuclei revealed by Hoechst staining, second the number of Casp3-ir cells and last the number of TH-ir perikarya of the dopaminergic A14 cell group. The A14 group was co-distributed with ERα-ir cells and was a marker of the PeV ( Fig. 6a ). The relatively constant number of TH-ir perikarya counted between sexes and across ages ( Fig. 6c ) ensured that a comparable tissue area was being sampled. The area considered the ‘PeV’ here was anatomically defined by the following landmarks: medially by the ependymal lining, laterally by the extension of the TH-ir catecholaminergic innervations from the brainstem and the distribution of the TH-ir somatodendritic profiles of the A14 group, dorsoventrally by the third ventricle and rostrocaudally by the anatomical planes of the two frontal slices harvested for culture (posterior to the foramen of Monroe and rostral to the A12 group). This periventricular continuum spans the anterior hypothalamic area and is thus clearly posterior to the distributional area of the A15 group in the periventricular preoptic hypothalamus [18] . All quantitative data are expressed as the mean±s.e.m. and were compared by two-way ANOVA or the Student’s t -test (as detailed in the figure legends) with significance set at P <0.05 (SigmaStat). How to cite this article: Israel, J.-M. et al. Neonatal testosterone suppresses a neuroendocrine pulse generator required for reproduction. Nat. Commun. 5:3285 doi: 10.1038/ncomms4285 (2014).